Transcriptional repression ofGIF1by the KIX-PPD-MYC repressor complex controls seed size in Arabidopsis Seed size is a key agronomic trait that greatly determines plant yield. Elucidating the molecular mechanism underlying seed size regulation is also an important question in developmental biology. Here, we show that the KIX-PPD-MYC-GIF1 pathway plays a crucial role in seed size control in Arabidopsis thaliana . Disruption of KIX8/9 and PPD1/2 causes large seeds due to increased cell proliferation and cell elongation in the integuments. KIX8/9 and PPD1/2 interact with transcription factors MYC3/4 to form the KIX-PPD-MYC complex in Arabidopsis. The KIX-PPD-MYC complex associates with the typical G-box sequence in the promoter of GRF - INTERACTING FACTOR 1 ( GIF1 ), which promotes seed growth, and represses its expression. Genetic analyses support that KIX8/9, PPD1/2, MYC3/4, and GIF1 function in a common pathway to control seed size. Thus, our results reveal a genetic and molecular mechanism by which the transcription factors MYC3/4 recruit KIX8/9 and PPD1/2 to the promoter of GIF1 and repress its expression, thereby determining seed size in Arabidopsis. Seed size is one of important agronomic traits that influences seed yield of crops, and elucidating the molecular mechanism underlying seed size control will help to improve seed yield. In flowering plants, a mature seed consists of the embryo, endosperm and seed coat. Seed development starts with double fertilisation. One sperm cell fuses with the egg cell to form the embryo, and another sperm cell fuses with the central cell to generate the endosperm. Thus, the embryo and endosperm are derived from the zygotic tissues. The seed coat, which envelops the embryo and the endosperm, is derived from maternal integuments [1] , [2] , [3] , [4] . Seed size is therefore coordinately determined by zygotic and maternal tissues. Several genes have been shown to control seed size in Arabidopsis thaliana , such as DA1 , ENHANCER OF DA1 - 1 ( EOD3 ), SUPPRESSOR OF DA1 - 1 ( SOD7 ), BIG BROTHER ( BB / EOD1 ), UBIQUITION - SPECIFIC PROTEIASE ( UBP15 ) GRF - INTERACTING FACTOR 1 ( GIF1 ), SAMBA , AUXIN RESPONSE FACTOR 2 ( ARF2 ), ARABIDOPSIS G PROTEIN GAMMA SUBUNIT 3 ( AGG3 ), APETALA 2 ( AP2 ), KLU and IKU1 / 2 [4] , [5] . However, the genetic and molecular mechanisms underlying seed size regulation are complicated and still largely unknown. Cell proliferation and cell growth coordinately determine the organ size during the plant organogenesis [6] , [7] . GRF-INTERACTING FACTORs (GIF1/2/3), a group of transcriptional co-activators, interact with Growth-Regulating Factors (GRFs) to control leaf, flower, and root development by regulating cell proliferation and growth [8] , [9] , [10] , [11] , [12] , [13] , [14] . The gif1 single mutants produce significantly smaller leaves and flowers than wild-type plants resulting from reduced cell number in Arabidopsis, while overexpression of GIF1 results in large leaf size due to an increase of cell number [8] , [9] , [10] , [11] , [13] . In addition, GIF1 also recruits SWI/SNF chromatin remodelling complexes to its target genes that can be transcriptionally activated or repressed by GRFs [15] . In rice, overexpression of OsGIF1 increases the size of leaves, stems, and grains, while loss-of-function of OsGIF1 leads to small plants [16] , [17] . In maize, gif1 mutants are dwarf with narrow leaves resulting from a less cell number [18] . GIFs are involved in many developmental processes, but the molecular mechanisms of transcription activation and inhibition of GIFs is unknown. PEAPODs (PPD1/2), which belong to the TIFY class II protein family, control leaf development, seed growth and germination, hypocotyl elongation, stomata development and flowering time [19] , [20] , [21] , [22] . Suppression of PPD genes leads to big and dome-shape leaves resulting from prolonged cell proliferation. PPD1/2 interact with KINASE-INDUCIBLE DOMAIN INTERACTING 8/9 (KIX8/9) and TOPLESS (TPL) to form a repressor protein complex, which controls the leaf development by influencing the expression of cell division-related genes [21] , [22] . The stability of KIX-PPD complex is regulated by an F-box protein STERILE APETALA (SAP) that acts as a part of the SKP1/Cullin/F-box E3 ubiquitin ligase complex [22] , [23] . SAP positively regulates organ growth by targeting the KIX-PPD complex for 26S proteasome-dependent degradation [22] , [23] . Here, we find that the KIX-PPD complex controls maternal integument development and influences seed size by regulating cell proliferation and growth. KIX8/9 and PPD1/2 interact with transcription factors MYC3/4 to form the KIX-PPD-MYC complex in Arabidopsis. The KIX-PPD-MYC complex binds to the typical G-box sequence in the GIF1 promoter and represses its expression. Genetic analyses show that GIF1 functions as a downstream factor of the SAP-KIX-PPD-MYC signalling pathway to control seed size. Our results reveal a genetic and molecular mechanism by which the transcriptional repression of GIF1 by the KIX-PPD-MYC complex regulates seed size in Arabidopsis. The KIX-PPD complex represses seed growth KINASE-INDUCIBLE DOMAIN INTERACTING 8/9 (KIX8/9) and PEAPOD1/2 (PPD1/2) were previously reported to form a KIX-PPD complex and regulate leaf size by influencing cell proliferation in Arabidopsis thaliana [21] , [22] . Here, we found an important function of the KIX-PPD complex in seed size control. The kix8 - 1 plants exhibited larger seeds than wild-type (Col-0) plants (Fig. 1 a, c). Seed weight of kix8 - 1 plants was also heavier than that of wild-type plants (Fig. 1d ). The size of cotyledons usually reflects changes in seed size [24] , [25] , [26] . Consistent with this, cotyledons of kix8 - 1 were larger than wild-type cotyledons (Fig. 1 b, e ). By contrast, seed size and weight and cotyledon area in kix9 - 1 plants were similar to those in the wild type (Fig. 1 a– e ). The kix8 - 1 kix9 - 1 double mutant showed significantly larger and heavier seeds and bigger cotyledons than the kix8 - 1 and kix9 - 1 single mutant (Fig. 1 a– e ), indicating that KIX8 and KIX9 function redundantly to control seed size and weight in Arabidopsis. Fig. 1: The KIX-PPD complex acts maternally to control seed development. a , b The seeds ( a ) and 8-day-old seedlings ( b ) of Col-0, kix8 - 1 , kix9 - 1 , kix8 - 1 kix9 - 1 , ppd1 - 2 , ppd2 - 1 , ppd1 - 2 ppd2 - cr , ppd1 - cr ppd2 - 1 , and kix8 - 1 kix9 - 1 ppd1 - 2 ppd2 - cr plants. c – e The relative seed area ( c , n = 100), 100 seed weight ( d , n = 10), and cotyledon area ( e , n = 30) of Col-0, kix8 - 1 , kix9 - 1 , kix8 - 1 kix9 - 1 , ppd1 - 2 , ppd2 - 1 , ppd1 - 2 ppd2 - cr , ppd1 - cr ppd2 - 1 , and kix8 - 1 kix9 - 1 ppd1 - 2 ppd2 - cr . Seeds from the third to seventh silique on the stem of six plants were used for analysis. Cotyledons from the 8-day-old seedlings were used for analysis. f , g The relative area of F 1 seeds ( f ) and F 2 seeds ( g ) from Col-0/Col-0 (C/C), Col-0/ kix8 - 1 kix9 - 1 ppd1 - 2 ppd2 - cr (C/kkpp), kix8 - 1 kix9 - 1 ppd1 - 2 ppd2 - cr /Col-0 (kkpp/C), and kix8 - 1 kix9 - 1 ppd1 - 2 ppd2 - cr / kix8 - 1 kix9 - 1 ppd1 - 2 ppd2 - cr (kkpp/kkpp) plants ( n = 100). h Ovules of Col-0 and kix8 - 1 kix9 - 1 ppd1 - 2 ppd2 - cr plants at 0 DAP (days after pollination). i – l The seed area ( i ), outer integument length ( j ), outer integument cell number ( k ), and outer integument cell length ( l ) of Col-0 and kix8 - 1 kix9 - 1 ppd1 - 2 ppd2 - cr plants at 0, 2, 4, and 6 DAP ( n = 33). Ovules and seeds from six siliques, which were from the fourth silique on the stem of six plants, were used for analysis. Scale bars, 0.5 mm ( a ), 0.2 cm ( b ), and 50 μm ( h ). Error bars represent ±SE. Different lowercase letters above the columns indicate the significant difference among different groups, one-way ANOVA P -values: P < 0.05. * indicates significant difference from the Col-0, one-way ANOVA P -values: * P < 0.05 and ** P < 0.01. Full size image Seed area and weight and cotyledon area in ppd2 - 1 plants were increased compared with those in wild-type plants, while seed area and weight and cotyledon area in ppd1 - 2 plants were comparable to those in wild-type plants (Fig. 1 a– e ). Because the PPD1 gene ( AT4G14713 ) is close to the PPD2 gene ( AT4G14720 ) in the chromosome, we could not isolate the ppd1 - 2 ppd2 - 1 double mutants. We generated ppd2 - cr mutation in the ppd1 - 2 mutant background and ppd1 - cr mutation in the ppd2 - 1 mutant background to obtain the ppd1 - 2 ppd2 - cr and ppd1 - cr ppd2 - 1 double mutants using the CRISPR-Cas9 technology, respectively (Supplementary Fig. 1 ) [27] . The ppd1 - 2 ppd2 - cr and ppd1 - cr ppd2 - 1 mutants had similar phenotypes (Fig. 1a – e ). Seed area and weight and cotyledon area in ppd1 - 2 ppd2 - cr and ppd1 - cr ppa2 - 1 mutants were significantly increased compared with those in ppd1 - 2 and ppd2 - 1 single mutants (Fig. 1 a– e ), indicating that PPD1 and PPD2 function redundantly to control seed size and weight. The ami - ppd and ppd2 - 1 plants have been reported to produce large and curvatured leaves with more cell number [19] , [20] , [21] . Interestingly, we observed that ppd1 - 2 ppd2 - cr and ppd1 - cr ppd2 - 1 showed strong curvature of leaves (Supplementary Fig. 2 a), indicating that ppd1 - 2 ppd2 - cr and ppd1 - cr ppd2 - 1 are strong alleles compared with ami - ppd . We measured the leaf area of 32-d-old Col-0, ppd1 - 2 ppd2 - cr and ppd1 - cr ppd2 - 1 plants and found that the third to eight leaves of ppd1 - 2 ppd2 - cr and ppd1 - cr ppd2 - 1 were smaller than those of wild type, but the tenth and eleventh leaves of ppd1 - 2 ppd2 - cr and ppd1 - cr ppd2 - 1 were larger than those of wild type (Supplementary Fig. 2 b, c). Considering that ami - ppd leaves had more cells than Col-0 leaves, we further examined palisade cell size and number of ppd1 - 2 ppd2 - cr and ppd1 - cr ppd2 - 1 fifth leaves. The palisade cell size of ppd1 - 2 ppd2 - cr and ppd1 - cr ppd2 - 1 plants was smaller than that of wild-type plants (Supplementary Fig. 2 d, e). By contrast, the palisade cell number in ppd1 - 2 ppd2 - cr and ppd1 - cr ppd2 - 1 leaves was higher than that in wild-type leaves (Supplementary Fig. 2 e), consistent with higher cell number in ami - ppd and ppd2 - 1 leaves [19] , [20] , [21] . These results supported that ppd1 - 2 ppd2 - cr and ppd1 - cr ppd2 - 1 promote cell proliferation in leaves, but decrease cell expansion. These data also suggest a possible compensation mechanism between cell number and cell size in ppd1 - 2 ppd2 - cr and ppd1 - cr ppd2 - 1 . This compensation phenomenon has been observed in several mutants [28] , [29] , [30] . Considering that KIX8/9 and PPD1/2 function in a complex [21] , [22] , we investigated the effect of simultaneous disruption of KIX8/9 and PPD1/2 on seed size. Seed area and weight and cotyledon area in the kix8 - 1 kix9 - 1 ppd1 - 2 ppd2 - cr quadruple mutant were similar to those of ppd1 - 2 ppd2 - cr or ppd1 - cr ppa2 - 1 double mutants (Fig. 1 a– e ) suggesting that KIX8/9 and PPD1/2 act in the common pathway to control seed size. Together, these results show that the KIX-PPD complex restricts seed growth in Arabidopsis. The KIX-PPD complex acts maternally to regulate seed size Seed size is determined coordinately by the growth of maternal and zygotic tissues [1] , [4] . To investigate whether the KIX-PPD complex functions maternally or zygotically to control seed size, we performed the reciprocal crossing experiments between the wild type and kix8 - 1 kix9 - 1 ppd1 - 2 ppd2 - cr . As shown in Fig. 1f , the F 1 seed area of Col-0 plants pollinated with the pollen of kix8 - 1 kix9 - 1 ppd1 - 2 ppd2 - cr plants was similar to that of self-pollinated Col-0 plants, and the F 1 seed area of kix8 - 1 kix9 - 1 ppd1 - 2 ppd2 - cr plants pollinated with the pollen of Col-0 plants was comparable to that of self-pollinated kix8 - 1 kix9 - 1 ppd1 - 2 ppd2 - cr plants. The size of Col-0/ kix8 - 1 kix9 - 1 ppd1 - 2 ppd2 - cr and kix8 - 1 kix9 - 1 ppd1 - 2 ppd2 - cr /Col-0 F 2 seeds was similar to that of Col-0/Col-0 F 2 seeds and smaller than that of kix8 - 1 kix9 - 1 ppd1 - 2 ppd2 - cr / kix8 - 1 kix9 - 1 ppd1 - 2 ppd2 - cr F 2 seeds (Fig. 1g ). In addition, reciprocal crossing experiments showed that kix8 - 1 or ppd2 - 1 single mutation acts maternally to influence seed size (Supplementary Fig. 3 ). Together, these results indicate that the KIX-PPD complex regulates seed growth through the maternal tissue of mother plants. As the integuments belong to maternal tissues in Arabidopsis, we investigated the development of the outer integuments in the wild type and kix8 - 1 kix9 - 1 ppd1 - 2 ppd2 - cr . The kix8 - 1 kix9 - 1 ppd1 - 2 ppd2 - cr plants had bigger ovule area and longer outer integuments than wild-type plants at 0 DAP (days after pollination) (Fig. 1 h–j). We then counted the number of cells in wild-type and kix8 - 1 kix9 - 1 ppd1 - 2 ppd2 - cr outer integuments and found that kix8 - 1 kix9 - 1 ppd1 - 2 ppd2 - cr outer integuments contained more cells than wild-type outer integuments (Fig. 1k ). By contrast, the length of cells in kix8 - 1 kix9 - 1 ppd1 - 2 ppd2 - cr outer integuments was similar to that in wild-type outer integuments (Fig. 1l ). These results indicate that the KIX-PPD module restricts cell proliferation in outer integuments before fertilisation. We then examined cell number and cell length in wild-type and kix8 - 1 kix9 - 1 ppd1 - 2 ppd2 - cr outer integuments at 2, 4 and 6 DAP, respectively. The outer integument cell number and cell length of kix8 - 1 kix9 - 1 ppd1 - 2 ppd2 - cr were increased compared with those of the wild type at 4 and 6 DAP (Fig. 1 k–l), thereby resulting in long outer integument and large seed size in the kix8 - 1 kix9 - 1 ppd1 - 2 ppd2 - cr plants (Fig. 1 i–j). These results indicate that the KIX-PPD module limits both cell proliferation and cell elongation in outer integuments after fertilisation. We further compared the effect of kix8 - 1 kix9 - 1 ppd1 - 2 ppd2 - cr on cell proliferation during ovule and seed developmental processes. As shown in Fig. 1k , the KIX-PPD module restrains cell proliferation of the outer integument during both ovule and early seed developmental stages. The formation of the KIX8/9-PPD1/2-MYC3/4 complex PPD1/2 and 12 JAZ proteins belong to TIFY class II protein family [31] . JAZ proteins usually interact with transcription factors to perform their functions, such as ENHANCER OF GLABRA 3 (EGL3), GLABROUS 3 (GL3), TRANSPARENT TESTA 8 (TT8), MYELOCYTOMATOSIS 2/3/4 (MYC2/3/4), MYB21/24, GLABRA 1 (GL1), PURPLE ACID PHOSPHATASE 1 (PAP1), ETHYLENE-INSENSITIVE 3 (EIN3) and ETHYLENE-INSENSITIVE3-LIKE 1 (EIL1) [32] , [33] , [34] , [35] . We therefore used the split luciferase complementation assays to test whether PPD proteins could interact with these transcription factors. We found that PPD1 and PPD2 interacted with MYC3 and MYC4 (Fig. 2a ), but not with MYC2 and other transcription factors (Supplementary Fig. 4 ). By contrast, we did not detect the interactions between KIX8/9 and MYC2/3/4 in split luciferase complementation assays (Supplementary Fig. 5 ). The interactions between PPD1/2 and MYC3/4 were further verified by forster resonance energy transfer and fluorescence lifetime imaging microscopy analyses (FRET-FLIM). As shown in Fig. 2b , the CFP fluorescence lifetime of MYC3-CFP was significantly decreased by the PPD1-YFP or PPD2-YFP in N. benthamiana leaves. The CFP fluorescence lifetime of MYC4-CFP was also significantly decreased by the PPD1-YFP or PPD2-YFP in N. benthamiana leaves. The bimolecular fluorescence complementation assays also showed that nYFP-PPD1 and nYFP-PPD2 associated with cYFP-MYC3 and cYFP-MYC4, but not with the cYFP control (Supplementary Fig. 6 ). To determine whether PPD1/2 could directly interact with MYC3/4 in vitro, we performed pull-down analyses. As shown in Fig. 2c , GST-MYC3/4 bound to MBP-PPD1/2 in vitro, but not the MBP control. Fig. 2: KIX8/9, PPD1/2, and MYC3/4 form a complex in Arabidopsis. a Split luciferase complementation assays showing the interactions between PPD1/2 and MYC3/4. MYC3/4-nLUC and cLUC-PPD1/2 were coexpressed in N. benthamiana leaves. The luciferase activity was detected at 2 days later after infiltration. b The FRET-FLIM assays showing that MYC3/4 interact with PPD1/2 in N. benthamiana leaves. CFP fluorescence lifetime was obtained at 2 days later after coinfiltrating with different combinations of 35S : MYC3 - CFP , 35S : MYC4 - CFP , 35S : PPD1 - YFP , 35S : PPD2 - YFP , and 35S : DEL1 - YFP constructs. 35S : DEL1 - YFP was used as a negative control. c Pull-down analyses showing the interactions between PPD1/2 and MYC3/4 in vitro. GST-MYC3 and GST-MYC4 were incubated with MBP-PPD1, MBP-PPD2, and MBP, respectively. Proteins were pulled down by MBP-Trap-A agarose beads and detected by Western blot with anti-GST or anti-MBP antibody. d Co-immunoprecipitation analyses showing the interactions between PPD1/2 and MYC3/4 in Arabidopsis. Total protein extracts of 35S : Myc - PPD1 / 2 ; 35S : GFP and 35S : Myc - PPD1 / 2 ; 35S : GFP - MYC3 / 4 plants were incubated with GFP-Trap agarose beads. Precipitates were detected by Western blot with anti-GFP or anti-Myc antibody. e Pull-down analyses showing that PPD1/2 are required for the interactions between KIX8 and MYC3/4. His-KIX8 was incubated with GST-MYC3 or GST-MYC4 and MBP-PPD1 or MBP-PPD2. Proteins were pulled down by the Ni-NTA agarose beads and detected by Western blot with anti-GST, anti-MBP, or anti-His antibody. f Co-immunoprecipitation analyses showing that KIX8/9 and MYC3/4 are in a protein complex in Arabidopsis. Total protein extracts of 35S : Myc - KIX8 / 9;35S : GFP and 35S : Myc - KIX8 / 9;35S : GFP - MYC3 / 4 plants were incubated with GFP-Trap agarose beads. Precipitates were detected by Western blot with anti-GFP or anti-Myc antibody. Full size image To investigate whether PPD1/2 could interact with MYC2/3/4 in Arabidopsis, we generated 35S : Myc - PPD1 #8, 35S : Myc - PPD2 #5, 35S : GFP - MYC2 #4, 35S : GFP - MYC3 #12, and 35S : GFP - MYC4 #8 transgenic lines. 35S : Myc - PPD1 #8, 35S : Myc - PPD2 #5, 35S : GFP - MYC3 #12, and 35S : GFP - MYC4 #8 transgenic lines produced small seeds (Supplementary Figs. 9 and 10 ), indicating that they are functional. We crossed 35S : Myc - PPD1 #8 and 35S : Myc - PPD2 #5 lines with 35S : GFP , 35S : GFP - MYC2 #4, 35S : GFP - MYC3 #12, and 35S : GFP - MYC4 #8 lines to generate 35S : Myc - PPD1 ; 35S : GFP , 35S : Myc - PPD1 ; 35S : GFP - MYC2 , 35S : Myc - PPD1 ; 35S : GFP - MYC3 , 35S : Myc - PPD1 ; 35S : GFP - MYC4 , 35S : Myc - PPD2 ; 35S : GFP , 35S : Myc - PPD2 ; 35S : GFP - MYC2 , 35S : Myc - PPD2 ; 35S : GFP - MYC3 and 35S : Myc - PPD2 ; 35S : GFP - MYC4 plants, respectively. Co-immunoprecipitation analyses (co-IP) showed that Myc-PPD1/2 associated with GFP-MYC3/4 but not with the GFP control (Fig. 2d ), indicating that PPD1/2 and MYC3/4 form a complex in Arabidopsis. The interactions between Myc-PPD1/2 and GFP-MYC2 were not found by co-immunoprecipitation analyses in Arabidopsis (Supplementary Fig. 7 ). Pull-down analyses showed that His-KIX8 could not directly associate with GST-MYC3/4 in vitro (Fig. 2e ). Considering that KIX8/9 can interact with PPD1/2 [21] , we incubated His-KIX8 with MBP-PPD1/2 and GST-MYC3/4. When proteins were pulled down by Ni-NTA agarose, we detected the MBP-PPD1/2 and GST-MYC3/4 proteins (Fig. 2e ), indicating that KIX8, PPD1/2, and MYC3/4 could form a complex in vitro. The associations of His-KIX9 with GST-MYC3/4 were not found in similar assays (Supplementary Fig. 8 ). To further investigate whether KIX8/9, PPD1/2, and MYC3/4 form a complex in Arabidopsis, we generated 35S : Myc - KIX8 #6 and 35S : Myc - KIX9 #14 transgenic lines that formed small seeds compared with the wild type (Supplementary Fig. 9 ), and crossed them with 35S : GFP , 35S : GFP - MYC3 #12, and 35S : GFP - MYC4 #8 plants to isolate 35S : Myc - KIX8 ; 35S : GFP , 35S : Myc - KIX8 ; 35S : GFP - MYC3 , 35S : Myc - KIX8 ; 35S : GFP - MYC4 , 35S : Myc - KIX9 ; 35S : GFP , 35S : Myc - KIX9 ; 35S : GFP - MYC3 and 35S : Myc - KIX9 ; 35S : GFP - MYC4 plants, respectively. Co-immunoprecipitation analyses revealed that Myc-KIX8/9 and GFP-MYC3/4 exist in a complex (Fig. 2f ). Together, these results indicate that KIX8/9, PPD1/2, and MYC3/4 form a KIX-PPD-MYC complex in Arabidopsis. MYC3 and MYC4 function redundantly to regulate seed size As MYC3/4 could interact with PPD1/2, we asked whether MYC3 / 4 influence seed size. As shown in Fig. 3 a–c, e, myc3 (GK_445B11) and myc4 (GK_491E10) plants produced larger seeds and cotyledons than the wild-type plants, consistent with a previous study [36] . The myc3 and myc4 plants also had heavier seed weight than the wild-type plants (Fig. 3d ). The myc3 myc4 double mutant produced larger and heavier and bigger cotyledons than myc3 and myc4 single mutant (Fig. 3 a–e), indicating that MYC3 and MYC4 function redundantly to regulate seed size and weight. In addition, overexpression of GFP-MYC3/4 fusion proteins driven by the CaMV 35S promoter in wild-type plants resulted in small and light seeds compared with the wild type (Supplementary Fig. 10 ), indicating that MYC3/4 limit seed growth in Arabidopsis. Fig. 3: MYC3 and MYC4 act maternally to control seed development. a , b The seeds ( a ) and 8-day-old seedlings ( b ) of Col-0, myc3 , myc4 , and myc3 myc4 . c – e The relative seed area ( c , n = 100), 100 seed weight ( d , n = 10), and cotyledon area ( e , n = 30) of Col-0, myc3 , myc4 and myc3 myc4 . Seeds from the third to seventh silique on the stem of six plants were used for analysis. Cotyledons from the 8-day-old seedlings were used for analysis. f , g The relative area of F 1 seeds ( f ) and F 2 seeds ( g ) from the Col-0/Col-0 (C/C), Col-0/ myc3 myc4 (C/mm), myc3 myc4 /Col-0 (mm/C), and myc3 myc4 / myc3 myc4 (mm/mm) plants (n = 100). h Ovules of Col-0 and myc3 myc4 plants at 0 DAP (days after pollination). i – l The seed area ( i ), outer integument length ( j ), outer integument cell number ( k ), and outer integument cell length ( l ) of Col-0 and myc3 myc4 plants at 0, 2, 4, and 6 DAP (n = 33). Ovules and seeds from six siliques, which were from the fourth silique on the stem of six plants, were used for analysis. Scale bars, 0.5 mm ( a ), 0.2 cm ( b ), and 50 μm ( h ). Error bars represent ±SE. Different lowercase letters above the columns indicate the significant difference among different groups, one-way ANOVA P -values: P < 0.05. * indicates significant difference from the Col-0, one-way ANOVA P -values: * P < 0.05 and ** P < 0.01. Full size image To investigate whether MYC3 / 4 function maternally or zygotically to control seed size, we performed reciprocal crossing experiments between the myc3 myc4 and wild type plants. As shown in Fig. 3f , the F 1 seed area of Col-0 plants pollinated with the pollen of myc3 myc4 plants was similar to that of self-pollinated Col-0 plants, and the F 1 seed area of myc3 myc4 plants pollinated with the pollen of Col-0 plants was comparable to that of self-pollinated myc3 myc4 plants. In addition, the size of Col-0/ myc3 myc4 and myc3 myc4 /Col-0 F 2 seeds was similar to that of Col-0/Col-0 F 2 seeds and smaller than that of myc3 myc4 / myc3 myc4 F 2 seeds (Fig. 3g ). These results indicate that MYC3 / 4 act maternally to control seed size. We then examined the development of wild-type and myc3 myc4 outer integuments. myc3 myc4 plants had larger ovules and longer outer integuments than the wild-type plants at 0 DAP (Fig. 3 h–j). The number of cells in myc3 myc4 outer integuments was increased compared with that in wild-type outer integuments, while the outer integument cell length of myc3 myc4 was similar to that of the wild type at 0 DAP (Fig. 3 k, l). These results indicate that MYC3 / 4 limit cell proliferation in the ovules before fertilisation. We further examined cell number and cell length in wild-type and myc3 myc4 outer integuments at 2, 4 and 6 DAP. The outer integument cell number and length of myc3 myc4 were significantly increased compared with those of the wild type at 4 and 6 DAP, thereby resulting in longer outer integument and larger seed size in the myc3 myc4 plants (Fig. 3 i–l). These results indicate that MYC3 / 4 limit both cell proliferation and cell elongation in outer integuments after fertilisation, consistent with the role of the KIX-PPD complex. We further compared the effect of myc3 myc4 on cell proliferation during ovule and seed developmental processes. As shown in Fig. 3k , MYC3 / 4 restrict cell proliferation in the integuments during both ovule and early seed developmental stages. The KIX-PPD-MYC complex represses GIF1 expression We previously reported the SAP-KIX-PPD signalling pathway has an important role in leaf size control [22] , [23] , and performed the RNA-seq analysis using the first pair of leaves of 9-day-old myc3 myc4 and ppd1 - 2 ppd2 - cr seedlings. 149 genes with significantly changed expression were found in both myc3 myc4 and ppd1 - 2 ppd2 - cr plants (Supplementary Data 1 ). One of them was the transcriptional coactivator GIF1 ( GRF - INTERACTING FACTOR 1 ), which has been reported to control the size of leaves, flowers, seeds, and cotyledons [8] , [9] , [10] , [11] , [13] , [37] , [38] . The expression of GIF1 was significantly upregulated in both myc3 myc4 and ppd1 - 2 ppd2 - cr seedlings (Supplementary Data 1 ). We also found that expression levels of GIF1 were significantly higher in kix8 - 1 kix9 - 1 , ppd1 - 2 ppd2 - cr , and myc3 myc4 siliques than those in wild-type siliques at 0, 2, and 4 DAF (days after flowering) (Fig. 4a ). By contrast, expression levels of GIF1 were decreased in the 2 DAF siliques of 35S : Myc - KIX 8 #6, 35S : Myc - KIX 9 #14, 35S : Myc - PPD1 #8, 35S : Myc - PPD2 #5, 35S : GFP - MYC3 #12, and 35S : GFP - MYC4 #8 plants compared with those of wild-type plants (Supplementary Fig. 11 ). In addition, the LUC activity of GIF1pro : LUC was significantly reduced by overexpressing Myc - KIX8 / 9 , Myc - PPD1 / 2 and Myc - MYC3 / 4 in the Col-0 protoplast (Fig. 4b ). These results indicate that the KIX-PPD-MYC complex represses GIF1 expression. The KIX-PPD module limits leaf development by the repressor TOPLESS (TPL) [21] , [22] . Overexpression of Myc-TPL also reduced the LUC activity of GIF1pro : LUC in the Col-0 protoplast (Fig. 4b ). Plant cis-acting regulatory DNA element analysis showed that there was a typical G-box sequence (5′-CACGTG-3′) at the -425 bp site in the 2 kb promoter region of GIF1 ( https://www.dna.affrc.go.jp/PLACE/?action=newplace ) (Fig. 4c ). MYCs and PPDs had been reported to associate with the G-box sequence to regulate target gene expression [21] , [39] . Furthermore, down-regulation of PPDs orthologs in legume Medicago truncatula and legume soybean leads to significant increases in expression of MtGIF1 and GmGIF1 [40] . These results imply that GIF1 might be a target gene of the KIX-PPD-MYC repressive complex. Fig. 4: The KIX-PPD-MYC complex associates with the promoter of GIF1 and represses its expression. a The relative expression levels of GIF1 in the 0, 2 and 4 DAF (days after flowering) siliques of Col-0, kix8 - 1 kix9 - 1 , ppd1 - 2 ppd2 - cr and myc3 myc4 were detected by qPCR ( n = 3). Data was normalised with ACTIN2 . b The LUC activity of GIF1pro : LUC from the transient expression analysis in the Col-0 and myc3 myc4 protoplast ( n = 5). GIF1pro : LUC was cotransfected with different combinations of 35S : Myc - KIX8 (K8), 35S : Myc - KIX9 (K9), 35S : Myc - PPD1 (P1), 35S : Myc - PPD2 (P2), 35S : Myc - MYC3 (M3), 35 S : Myc - MYC4 (M4), and 35S : Myc - TPL (TPL) into the Col-0 and myc3 myc4 protoplast. The LUC and REN luciferase activities of GIF1pro : LUC were measured 40 h later after transfection. NC ( pGreen II_0800 - LUC ) was used as a negative control. c The schematic diagram of GIF1 promoter containing a typical G-box (5′-CACGTG-3′) sequence in F1 fragment. F1 - F4 represent DNA fragments used for ChIP-qPCR analysis. d ChIP-qPCR assays showing that KIX8/9 and PPD1/2 associate with the promoter of GIF1 by MYC3/4 in Arabidopsis ( n = 4). Chromatin from 1 to 4 DAF siliques of 35S : GFP , 35S : GFP - MYC3 ; myc3 , 35S : GFP - MYC4 ; myc4 , 35S:GFP-MYC3;myc3 ppd1 - 2 ppd2 - cr , 35S : GFP - MYC4 ; myc4 ppd1 - 2 ppd2 - cr , 35S : GFP - MYC3 ; myc3 kix8 - 1 kix9-1 , 35S : GFP - MYC4 ; myc4 kix8 - 1 kix9-1 , 35S : GFP - PPD1 ; ppd1 - 2 , 35S : GFP - PPD2 ; ppd2 - 1 , 35S : GFP - PPD1 ; ppd1 - 2 myc3 myc4 , 35S : GFP - PPD2 ; ppd2 - 1 myc3 myc4 , 35S : GFP - KIX8 ; kix8 - 1 , 35S : GFP - KIX9 ; kix9 - 1 , 35S : GFP - KIX8 ; kix8 - 1 myc3 myc4 and 35S : GFP - KIX9 ; kix9 - 1 myc3 myc4 were incubated with ChIP anti-GFP antibody and precipitated by ChIP protein A + G magnetic beads. The enrichment of fragments was determined by qPCR. The 35S : GFP plants acted as a control. The ACTIN7 promoter was used as a negative control. e The sequence of A and A - m probes for EMSA analysis. f , g The associations of MBP-MYC3 ( g ) and MBP-MYC4 ( i ) with the promoter of GIF1 were detected by EMSA. 5′-biotin- A / A - m probes were incubated with MBP or MBP-MYC3/4 and detected by ChIP western blot with the anti-biotin antibody. Error bars represent ±SE. Asterisk indicates significant difference, one-way ANOVA P -values: ** P < 0.01. Different lowercase letters above the columns indicate the significant difference among different groups, one-way ANOVA P -values: P < 0.05. Full size image To test this possibility, we performed the chromatin immunoprecipitation-quantitative PCR (ChIP-qPCR) assays using the 1–4 DAF siliques of 35S : GFP , 35S : GFP - MYC3 ; myc3 , and 35S : GFP - MYC4 ; myc4 plants. The 35S : GFP - MYC3 ; myc3 and 35S : GFP - MYC4 ; myc4 plants formed small seeds compared with the wild type, indicating GFP-MYC3 and GFP-MYC4 are functional (Supplementary Fig. 12 ). As shown in Fig. 4 c, d, the fragment F1 from the GIF1 promoter containing the typical G-box cis-acting element in 35S : GFP - MYC3 ; myc3 and 35S : GFP - MYC4 ; myc4 plants was remarkably enriched compared with that in 35S : GFP plants. The fragment F1 from the GIF1 promoter was also significantly enriched compared with other fragments ( F2 - F4 ) without the typical G-box element and the negative control (a fragment of ACTIN7 promoter) in 35S : GFP - MYC3 ; myc3 and 35S : GFP - MYC4 ; myc4 plants, indicating that MYC3 and MYC4 associate with the GIF1 promoter through the fragment F1 in Arabidopsis. We then asked whether KIX8/9 and PPD1/2 could influence the associations of MYC3 and MYC4 with the GIF1 promoter. In 35S : GFP - MYC3 ; myc3 kix8 - 1 kix9 - 1 , 35S : GFP - MYC4 ; myc4 kix8 - 1 kix9 - 1 , 35S : GFP - MYC3 ; myc3 ppd1 - 2 ppd2 - cr and 35S : GFP - MYC4 ; myc4 ppd1 - 2 ppd2 - cr plants, the enrichment of F1 fragments was substantially decreased compared with that in 35S : GFP - MYC3 ; myc3 and 35S : GFP - MYC4 ; myc4 plants (Fig. 4d ), indicating that KIX8/9 and PPD1/2 are required for MYC3/4 to effectively bind to the GIF1 promoter. The fragment F1 from the GIF1 promoter in 35S : GFP - KIX8 ; kix8 - 1 , 35S : GFP - KIX9 ; kix9 - 1 , 35S : GFP - PPD1 ; ppd1 - 2 , and 35S : GFP - PPD2 ; ppd2 - 1 plants also could be strongly enriched compared with that in the 35S : GFP plants, while it could not be enriched in 35S : GFP - KIX8 ; kix8 - 1 myc3 myc4 , 35S : GFP - KIX9 ; kix9 - 1 myc3 myc4 , 35S : GFP - PPD1 ; ppd1 - 2 myc3 myc4 , and 35S : GFP - PPD2 ; ppd2 - 1 myc3 myc4 plants (Fig. 4d ). These results indicate that MYC3/4 are required for KIX8/9 and PPD1/2 to bind to the GIF1 promoter and repress its expression. Consistent with this, the LUC activity of GIF1pro : LUC was not reduced by the overexpression of Myc-KIX8/9, Myc-PPD1/2, and Myc-TPL driven by the CaMV 35S promoter in the myc3 myc4 protoplast (Fig. 4b ). To investigate whether MYC3/4 could directly bind to the G-box cis-acting element in the promoter of GIF1 , we performed the electrophoretic mobility shift assays (EMSA). As shown in Fig. 4 e–g, MBP-MYC3 and MBP-MYC4 bound to the biotin-labelled probe A from the GIF1 promoter containing the typical G-box (5′-CACGTG-3′) but not to the mutated biotin-labelled probe A ( A - m ). The binding ability of MBP-MYC3 and MBP-MYC4 to the probe A was decreased by adding the biotin-unlabelled probe A . These results indicate that MYC3 and MYC4 directly bind to the GIF1 promoter. GIF1 acts maternally to control seed size The gif1 plants (SALK_150407) produced smaller leaves, seeds, and cotyledons than wild-type plants (Fig. 5 a–c, e, and Supplementary Fig. 13 a), consistent with previous studies [8] , [10] , [11] . The seed weight of gif1 plants was also significantly lower than that of wild-type plants (Fig. 5d ). In addition, the fertility of gif1 plants was lower than that of wild-type plants (Supplementary Fig. 13 b). By contrast, overexpression of GIF1 ( 35S : GIF1 ) led to bigger and heavier seeds and bigger cotyledons than the wild type (Fig. 5 a–e). These results indicate that GIF1 is required for normal seed and other organs development. Fig. 5: GIF1 acts maternally to control seed development. a , b The seeds ( a ) and 8-day-old seedlings ( b ) of Col-0, gif1 , 35S : GIF1 # 4, and 35 S : GIF1 # 7. c – e The relative seed area ( c , n = 100), 100 seed weight ( d , n = 10), and cotyledon area ( e , n = 30) of Col-0, gif1 , 35S : GIF1 # 4, and 35S : GIF1 # 7. Seeds from the third to seventh silique on the stem of six plants were used for analysis. Cotyledons from the 8-day-old seedlings were used for analysis. f , g The relative area of F 1 seeds ( f ) and F 2 seeds ( g ) from Col-0/Col-0 (C/C), Col-0/ gif1 (C/g), gif1 /Col-0 (g/C), and gif1 / gif1 (g/g) plants ( n = 100). h The Mature ovule of Col-0 and gif1 plants at 0 DAP (days after pollination). i – l The seed area ( i ), outer integument length ( j ), outer integument cell number ( k ), and outer integument cell length ( l ) of Col-0 and gif1 plants at 0, 2, 4, and 6 DAP (n = 33). Ovules and seeds from six siliques, which were from the fourth silique on the stem of six plants, were used for analysis. Scale bars, 0.5 mm ( a ), 0.2 cm ( b ), and 50 μm ( h ). Error bars represent ±SE. Different lowercase letters above the columns indicate the significant difference among different groups, one-way ANOVA P -values: P < 0.05. Asterisk indicates significant difference from the Col-0, one-way ANOVA P -values: * P < 0.05 and ** P < 0.01. Full size image To investigate whether GIF1 functions maternally or zygotically to control seed size, we conducted reciprocal crossing experiments between the wild type and gif1 . As shown in Fig. 5f , the F 1 seed size of Col-0 plants pollinated with the pollen of gif1 plants was similar to that of self-pollinated Col-0 plants, and the F 1 seed size of gif1 plants pollinated with the pollen of Col-0 plants was comparable to that of self-pollinated gif1 plants. In addition, the size of Col-0/ gif1 and gif1 /Col-0 F 2 seeds was similar to that of Col-0/Col-0 F 2 seeds and bigger than that of gif1 / gif1 F 2 seeds (Fig. 5g ). These results support that GIF1 acts maternally to control seed size. We then investigated the outer integument cell number and cell length before and after fertilisation. The gif1 plants had shorter outer integuments with fewer and shorter cells than the wild type at 0 DAP (Fig. 5 h, j–l). We further examined the outer integument cell number and cell length after fertilisation. The gif1 showed shorter outer integuments and smaller seeds than the wild type before 6 DAP (Fig. 5 i, j). The outer integument cell number of gif1 was significantly decreased compared with that of the wild type at 2, 4 and 6 DAP (Fig. 5k ). The cells in gif1 outer integuments were shorter than those in wild-type outer integuments at 2 DAP, while they were longer than those in wild-type outer integuments at 6 DAP (Fig. 5l ), suggesting a compensation phenomenon between cell proliferation and cell elongation [28] , [41] , [42] . In addition, we observed that gif1 decreases cell proliferation in outer integuments during both ovule and early seed developmental stages (Fig. 5k ). Partially overlapping expression of KIX-PPD-MYC As KIX8 , KIX9 , PPD1 , PPD2 , MYC3 , MYC4 and GIF1 function in a signalling pathway to regulate seed size, we asked whether they have the similar expression patterns during ovule and seed development. To test this, we generated the KIX8pro : KIX8 - GFP , KIX9pro : KIX9 - GFP , PPD1pro : PPD1 - GFP , PPD2pro : PPD2 - GFP , MYC3pro : MYC3 - GFP , MYC4pro : MYC4 - GFP , and GIF1pro : GIF1 - GFP transgenic lines. As shown in Fig. 6 and Supplementary Fig. 14 , KIX8, KIX9, PPD1, PPD2, MYC3, MYC4, and GIF1 expressed in the integument and chalazal region of ovules before fertilisation. As shown in Fig. 6 , PPD1, KIX9 and GIF1 strongly expressed in the nuclei of outer integument cells before 2 DAP and became weak from 3 DAP during seed development. MYC4 strongly expressed in the nuclei of outer integument cells before 3 DAP and became weak from 4 DAP during seed development. PPD2, KIX8, and MYC3 expressed in the nuclei of outer integument cells before 6 DAP. As shown in Supplementary Fig. 14 , PPD1, KIX9 and GIF1 also expressed in the chalazal domain cells of seeds before 2 DAP and were not observed at 4 DAP. KIX8, PPD2, MYC3, and MYC4 expressed in the chalazal domain cells of seeds before 4 DAP. In addition, MYC3 and GIF1 expressed in endosperms before 4 DAP. These results indicate that KIX8 , KIX9 , PPD1 , PPD2 , MYC3 , MYC4 and GIF1 have overlapped expression patterns during ovule development and possess partially overlapped expression patterns during seed development, supporting that they function in a common pathway to control seed size. Moreover, the GFP fluorescence in the epidermal cells of GIF1pro : GIF1 - GFP ; myc3 myc4 outer integuments was observed at 4 and 5 DAP, which was not observed in GIF1pro : GIF1 - GFP plants (Fig. 6 ), supporting that MYC3/4 repress GIF1 expression. Fig. 6: Expression patterns of KIX8 , KIX9 , PPD1 , PPD2 , MYC3 , MYC4 , and GIF1 in epidermal cells of the outer integuments during seed development. The promotors of KIX8 (2,087 bp), KIX9 (1,714 bp), PPD1 (1,797 bp), PPD2 (2,153 bp), MYC3 (2,180 bp), MYC4 (2,132 bp), and GIF1 (2,337 bp) and their CDSs were cloned into the pMDC107 - GFP vector to generate KIX8pro : KIX8 - GFP , KIX9pro : KIX9 - GFP , PPD1pro : PPD1 - GFP, PPD2pro : PPD2 - GFP , MYC3pro : MYC3 - GFP , MYC4pro : MYC4 - GFP , and GIF1pro : GIF1 - GFP constructs, respectively. GFP fluorescence from the outer integuments of seeds was observed during seed development. DAP days after pollination. Scale bars = 25 μm. Full size image GIF1 acts with the KIX-PPD-MYC module to control seed size As the KIX-PPD-MYC complex associates with the promoter of GIF1 through MYC3/4 and represses its expression, we asked whether GIF1 act in a common pathway with the KIX-PPD-MYC module to control seed size. We crossed gif1 with myc3 myc4 , kix8 - 1 kix9 - 1 , and ppd1 - 2 ppd2 - cr to generate gif1 myc3 myc4 , gif1 kix8 - 1 kix9 - 1 , and gif1 ppd1 - 2 ppd2 - cr triple mutants, respectively. As shown in Fig. 7 a–c, e , the gif1 mutation entirely suppressed the large seed and cotyledon phenotypes of myc3 myc4 , indicating that gif1 is epistatic to myc3 myc4 with respect to seed and cotyledon size. Similarly, gif1 is also epistatic to myc3 myc4 with respect to seed weight (Fig. 7d ). The large size of seeds and cotyledons of kix8 - 1 kix9 - 1 and ppd1 - 2 ppd2 - cr plants was strongly but not entirely suppressed by the gif1 mutation (Fig. 7 a–c, e), indicating that KIX8/9 and PPD1/2 are strongly but not entirely dependent on GIF1 to control seed size. Similarly, the gif1 mutation strongly but not entirely suppressed the seed weight phenotype of kix8 - 1 kix9 - 1 and ppd1 - 2 ppd2 - cr plants (Fig. 7d ). These genetic analyses indicate that GIF1 acts in a common pathway with the KIX-PPD-MYC module to control seed size and weight. Fig. 7: GIF1 acts genetically with the KIX-PPD-MYC complex to control seed size. a , b The seeds ( a ) and 8-day-old seedlings ( b ) of Col-0, gif1 , myc3 myc4 , gif1 myc3 myc4 , kix8 - 1 kix9 - 1 , gif1 kix8 - 1 kix9 - 1 , ppd1 - 2 ppd2 - cr , gif1 ppd1 - 2 ppd2 - cr , 35S : SAP , and 35S:SAP ; gif1 plants. c – e The relative seed area ( c , n = 100), 100 seed weight ( d , n = 10), and cotyledon area ( e , n = 30) of Col-0, gif1 , myc3 myc4 , gif1 myc3 myc4 , kix8 - 1 kix9 - 1 , gif1 kix8 - 1 kix9 - 1 , ppd1 - 2 ppd2 - cr , gif1 ppd1 - 2 ppd2 - cr , 35S : SAP , and 35S:SAP ; gif1 plants. f The TPL-KIX-PPD-MYC complex associates with the G-box sequence of GIF1 promoter and represses its expression. g The transcriptional repression of GIF1 is relieved by SAP modulating the KIX-PPD module for 26S proteasome degradation. Without the KIX-PPD complex, the binding ability of MYC3/4 with the promoter of GIF1 is decreased and the GIF1 expression is increased. Seeds from the third to seventh silique on the stem of six plants were used for analysis. Cotyledons from the 8-day-old seedlings were used for analysis. Scale bars, 0.5 mm ( a ) and 0.2 cm ( b ). Error bars represent ±SE. Different lowercase letters above the columns indicate the significant difference among different groups, one-way ANOVA P -values: P < 0.05. Full size image The ppd1 - 2 ppd2 - cr and kix8 - 1 kix9 - 1 plants produced wider siliques than wild-type plants. By contract, gif1 plants had narrower siliques than wild-type plants (Supplementary Fig. 15 ). The gif1 mutation entirely suppressed the wide silique phenotype of kix8 - 1 kix9 - 1 plants and strongly suppressed the wide silique phenotype of ppd1 - 2 ppd2 - cr plants (Supplementary Fig. 15 ). In addition, the silique phenotype of gif1 myc3 myc4 was similar to that of gif1 (Supplementary Fig. 15 ). These genetic analyses indicate that GIF1 acts genetically with the KIX-PPD-MYC module to control silique development. The gif1 and ppd1 - 2 ppd2 - cr plants had lower fertility than wild-type plants (Supplementary Fig. 16 ). The myc3 myc4 and kix8 - 1 kix9 - 1 had similar fertility to wild-type plants, but the fertility of gif1 myc3 myc4 and gif1 kix8 - 1 kix9 - 1 was similar to that of gif1 plants (Supplementary Fig. 16 ). Additionally, the gif1 mutation decreased the fertility of ppd1 - 2 ppd2 - cr plants (Supplementary Fig. 16 ). All of the genetic analyses indicate that GIF1 acts with the KIX-PPD-MYC module to control multiple biological processes. GIF1 and SAP function in a common pathway to control seed size STERILE APETALA (SAP/SUPPRESSOR OF DA1, SOD3) acts as a part of the E3 ubiquitin ligase complex to control organ size by regulating the stability of the KIX-PPD complex [22] , [23] . The sod3 - 1 mutants produce small leaves, while 35S : SAP plants have large leaves [22] , [23] . We found that 35S : SAP plants also produced bigger seeds and cotyledons than the wild-type plants (Fig. 7 a–c, e). Similarly, 35S : SAP plants produced heavier seeds than wild-type plants (Fig. 7d ). The gif1 mutation strongly suppressed the large seed and cotyledon phenotype of 35S : SAP plants (Fig. 7 a–c, e). The gif1 mutation also strongly suppressed the heavy seed phenotype of 35S : SAP plants (Fig. 7d ). Additionally, 35S : SAP plants produced wider siliques than wild-type plants, while it was significantly suppressed by the gif1 mutation (Supplementary Fig. 15 ). Although 35S : SAP plants had similar fertility to wild-type plants, the fertility of 35S : SAP ; gif1 plants was similar to that of gif1 (Supplementary Fig. 16 ). Moreover, the GIF1 expression was obviously higher in the 3 DAP siliques of 35S : SAP plants than that in wild-type plants (Supplementary Fig. 17 ). These data indicate that GIF1 acts as a downstream factor of SAP to control seed size. Seed size is the key agronomic trait that greatly determines the grain yield of plants. Although several factors have been reported to affect seed size in plants [4] , [5] , the genetic and molecular mechanisms that determine seed size remain elusive. In this study, we discover a genetic and molecular mechanism that the transcription factors MYC3/4 recruit the repressor complex KIX8/9-PPD1/2 to the promoter of GIF1 and repress its expression, thereby determining seed size in Arabidopsis. Previous studies reported that PPD1 and PPD2 act redundantly to regulate leaf size and shape by influencing both the primary and the secondary mitotic arrest fronts [20] , [21] , [23] . Considering that ppd2 - 1 had large seeds, while ppd1 - 2 did not obviously affect seed size, ppd1 - 2 ppd2 - 1 double mutant will help understand the role of PPD1 / 2 in seed size control. However, the PPD1 gene ( AT4G14713 ) is close to the PPD2 gene ( AT4G14720 ) in the chromosome, we could not isolate ppd1 - 2 ppd2 - 1 double mutant. We therefore generated the ppd2 - cr mutation in the ppd1 - 2 mutant background and the ppd1 - cr mutation in the ppd2 - 1 mutant background to obtain the ppd1 - 2 ppd2 - cr and ppd1 - cr ppd2 - 1 double mutants using the CRISPR-Cas9 technology, respectively (Supplementary Fig. 1 ) [27] . The ppd1 - 2 ppd2 - cr and ppd1 - cr ppa2 - 1 mutants produced larger and heavier seeds than ppd1 - 2 and ppd2 - 1 single mutants (Fig. 1 a, c, d), indicating that PPD1 and PPD2 function redundantly to control seed size and weight. KIX8/9 interact with PPD1/2 to form a transcriptional repressor complex and control leaf size [21] , [22] . However, it is unclear whether the KIX-PPD complex affects seed growth in Arabidopsis. Here, we found that kix8 - 1 kix9 - 1 ppd1 - 2 ppd2 - cr plants produced significantly larger seeds than the wild type (Fig. 1 a, c). Reciprocal crossing experiments showed that the KIX-PPD complex functions maternally to control seed size (Fig. 1 f, g). Cellular observation indicated that the KIX-PPD complex predominantly represses cell proliferation and also slightly limiting cell elongation in the integuments (Fig. 3 k, l). These results reveal that the KIX-PPD complex negatively regulates seed growth in Arabidopsis. The transcriptional repressor complex usually interacts with the transcription factors to regulate gene expression [43] , [44] . We found that PPD1/2 could directly interact with the transcription factors MYC3/4 in vitro and in vivo, but not interact with MYC2. Although MYC3 and MYC4 share lots of overlapping functions with MYC2, distinct functions among them have been reported. For instance, MYC3 and MYC4 recognise similar cis -acting sequences (i.e. G-box and its variants) to MYC2, while the DNA-binding affinity of MYC3 and MYC4 differs from that of MYC2. MYC2 and MYC4 but not MYC3 interact with the JAZ4 protein. The expression levels of VEGETATIVE STORAGE PROTEIN 2 ( VSP2 ) and PLANT DEFENSIN 1.2 ( PDF1.2 ), two of JA marker genes, are significantly different in myc2 , myc3 , and myc4 single mutants when treated with JA [33] , [34] , [45] . We further reveal that KIX8/9, PPD1/2, and MYC3/4 can form a complex in Arabidopsis (Fig. 2 ). Like kix8 - 1 kix9 - 1 and ppd1 - 2 ppd2 - cr mutants, myc3 myc4 mutants produced bigger seeds than the wild type (Fig. 3 a, c), consistent with a previous study [36] , further suggesting that MYC3/4 have the overlapped function with KIX8/9 and PPD1/2 in seed size control. Reciprocal crossing experiments indicate that MYC3/4 act maternally to limit seed growth. Cellular observations show that MYC3/4 influence both cell proliferation and cell elongation in the integuments, consistent with the role of the KIX-PPD complex in seed growth control. Therefore, the KIX-PPD-MYC module is crucial for seed size control in Arabidopsis. To identify the targets of the KIX-PPD-MYC module in seed growth, we performed the RNA-seq and found that PPD1/2 and MYC3/4 repress the expression of GIF1 . The expression levels of GIF1 in 0, 2, and 4 DAF siliques from kix8 - 1 kix9 - 1 , ppd1 - 2 ppd2 - cr and myc3 myc4 plants were significantly higher than those of wild-type plants (Fig. 4a ). Consistent with this, overexpression of Myc-KIX8/9, Myc-PPD1/2, Myc-MYC3/4, and Myc-TPL could reduce the activity of GIF1pro : LUC (Fig. 4b ). In addition, EMSA experiments showed that MYC3 and MYC4 directly bind to the G-box sequence in the promoter of GIF1 (Fig. 4 f, g). ChIP-qPCR analyses showed that KIX8/9 and PPD1/2 associate with the promoter of GIF1 through MYC3/4 (Fig. 4d ). These findings indicate that MYC3/4 may recruit the transcriptional repressor complex TPL-KIX-PPD to the promoter of GIF1 to repress its expression (Fig. 7f ). Overexpression of KIX8 , KIX9 , PPD1 , PPD2 , MYC3 , or MYC4 led to small seeds (Supplementary Figs. 5 and 6 ), consistent with the result of PPD1OE ( PPDOE ) [19] . It is possible that overexpression of KIX8 , KIX9 , PPD1 , PPD2 , MYC3 , or MYC4 in Arabidopsis might have more probability to form the TPL-KIX-PPD-MYC complex that represses the expression of GIF1 , thereby resulting in small seeds. Interestingly, MYC proteins recruit the TPL-NINJIA-JAZ transcriptional repressor complex to regulate gene expression [43] , [46] , [47] . Overexpression of JAZ13 alone attenuates JA-induced defence responses in Arabidopsis leaves. Overexpression of NINJIA promotes root length when treated with MeJA [43] . Overexpression of MYC2, MYC3, or MYC4 accelerates JA-induced leaf senescence [46] . These results indicate that overexpression of the single complex components can cause phenotypes. The expression of GIF2 and GIF3 in the 3 DAP siliques of kix8 - 1 kix9 - 1 , ppd1 - 2 ppd2 - cr , and myc3 myc4 plants was also upregulated compared with that in the wild type (Supplementary Fig. 18 ). Down-regulation of PPDs orthologs in legume Medicago truncatula and legume soybean leads to high expression of MtGIF1 and GmGIF1 in leaves, stipules, and seeds, respectively [40] . These results indicate that the expression of GIFs regulated by PPDs might be a common mechanism in dicotyledon plants. The loss-of-function mutation in GIF1 produced smaller seeds and cotyledons than the wild type (Fig. 5 a–c, e), consistent with previous studies [10] , [11] . The gif1 mutant has fewer cells and longer cells in the integuments than the wild type (Fig. 5 k, l), suggesting a compensation mechanism between cell proliferation and cell elongation. This phenomenon has been observed in several seed size mutants [28] , [41] , [42] . In addition, GIF1 was reported to play significant roles in leaf, flower, and root development in Arabidopsis [8] , [9] , [10] , [11] , [12] , [13] , [14] , indicating that GIF1 is required for normal plant organ growth. Surprisingly, a previous study showed that one mutant allele of GIF1 ( an3 ) promotes seed growth [48] . In this study, we have sufficient evidence to support that GIF1 is a positive regulator of seed size in Arabidopsis. For example, loss-of-function of GIF1 formed small seeds, while overexpression of GIF1 produced large seeds (Fig. 5 a, c). The gif1 mutation completely suppresses the large and heavy seed phenotypes of myc3 myc4 (Fig. 7 c, d). By contrast, the gif1 mutation strongly but not entirely suppresses the seed size and weight phenotypes of kix81 - 1 kix91 - 1 and ppd1 - 2 ppd2 - cr (Fig. 7 c, d), implying that KIX8 / 9 and PPD1 / 2 might have other mechanisms that act independently of GIF1 to control seed development. These genetic analyses also reveal that GIF1 functions in a common pathway with the KIX-PPD-MYC module to control seed size in Arabidopsis. Consistent with this, KIX8 , KIX9 , PPD1 , PPD2 , MYC3 , MYC4 and GIF1 have overlapped expression patterns during ovule development and possess partially overlapped expression patterns during early seed developmental stages (Fig. 6 and Supplementary Fig. 14 ). STERILE APETALA (SAP/SUPPRESSOR OF DA1, SOD3) acts as a part of the E3 ubiquitin ligase complex to control organ size by regulating the stability of the PPD-KIX complex [22] , [23] . The expression of GIF1 was obviously higher in 35S : SAP plants than that in wild-type plants (Supplementary Fig. 17 ), indicating that the transcriptional repression of GIF1 is released by the F-box protein SAP that modulates the KIX-PPD complex for 26S proteasome degradation (Fig. 7g ). However, SAP did not modulate the stability of MYC3/4 proteins (Supplementary Fig. 19 ). Without the KIX-PPD complex, MYC3/4 could bind to the promoter of GIF1 , but the binding ability is significantly decreased (Fig. 4d ). Genetic analyses showed that the gif1 mutation strongly suppresses the large and heavy seed phenotypes of 35S : SAP (Fig. 7 c, d), suggesting that SAP and GIF1 act in a common pathway to regulate seed growth. Based on these genetic and biochemical analyses, we build up a genetic and molecular framework for the SAP-KIX-PPD-MYC-GIF1 module-mediated control of seed size and weight in Arabidopsis (Fig. 7 f, g). Seed size is one of the important targets for plant breeding. In this study, we found that the KIX-PPD-MYC-GIF1 pathway is crucial for seed size control in Arabidopsis. Interestingly, loss-of-function of PPD orthologs in legume Medicago truncatula and legume soybean increases seed size and weight as well as leaf size [40] . In pea, mutations in the PPD ortholog ELEPHANT-EAR-LIKE LEAF 1 or the KIX ortholog BIGGER ORGANS cause large flowers and leaves [49] . In rice, overexpression of OsGIF1 results in large grains, leaves, and stems, while suppression of OsGIF1 leads to small grains and organs [16] , [17] . These findings suggest that the KIX-PPD-MYC-GIF1 pathway may possess a conserved function in different plant species. Thus, it will be interesting to investigate the roles of the KIX-PPD-MYC-GIF1 pathway in crops and utilise their homologues to improve seed size in key crops. Plant material and growth conditions All of the mutants and transgenic plants were in Arabidopsis thaliana Col-0 ecotype. 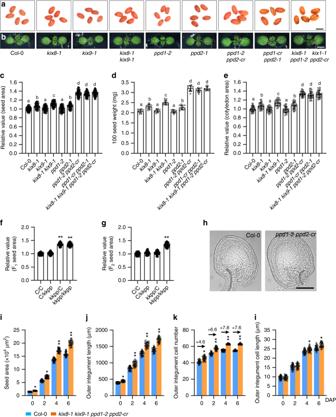Fig. 1: The KIX-PPD complex acts maternally to control seed development. a,bThe seeds (a) and 8-day-old seedlings (b) of Col-0,kix8-1,kix9-1,kix8-1 kix9-1,ppd1-2,ppd2-1,ppd1-2 ppd2-cr,ppd1-cr ppd2-1, andkix8-1 kix9-1 ppd1-2 ppd2-crplants.c–eThe relative seed area (c,n= 100), 100 seed weight (d,n= 10), and cotyledon area (e,n= 30) of Col-0,kix8-1,kix9-1,kix8-1 kix9-1,ppd1-2,ppd2-1,ppd1-2 ppd2-cr,ppd1-cr ppd2-1, andkix8-1 kix9-1 ppd1-2 ppd2-cr. Seeds from the third to seventh silique on the stem of six plants were used for analysis. Cotyledons from the 8-day-old seedlings were used for analysis.f,gThe relative area of F1seeds (f) and F2seeds (g) from Col-0/Col-0 (C/C), Col-0/kix8-1 kix9-1 ppd1-2 ppd2-cr(C/kkpp),kix8-1 kix9-1 ppd1-2 ppd2-cr/Col-0 (kkpp/C), andkix8-1 kix9-1 ppd1-2 ppd2-cr/kix8-1 kix9-1 ppd1-2 ppd2-cr(kkpp/kkpp) plants (n= 100).hOvules of Col-0 andkix8-1 kix9-1 ppd1-2 ppd2-crplants at 0 DAP (days after pollination).i–lThe seed area (i), outer integument length (j), outer integument cell number (k), and outer integument cell length (l) of Col-0 andkix8-1 kix9-1 ppd1-2 ppd2-crplants at 0, 2, 4, and 6 DAP (n= 33). Ovules and seeds from six siliques, which were from the fourth silique on the stem of six plants, were used for analysis. Scale bars, 0.5 mm (a), 0.2 cm (b), and 50 μm (h). Error bars represent ±SE. Different lowercase letters above the columns indicate the significant difference among different groups, one-way ANOVAP-values:P< 0.05. * indicates significant difference from the Col-0, one-way ANOVAP-values: *P< 0.05 and **P< 0.01. The seeds of ppd1 - 2 (SALK_057237), ppd2 - 1 (SALK_142698), kix8 - 1 (GABI_422H04), kix9 - 1 (SAIL_1168_G09), gif1 (SALK_150407), myc3 (GK_445B11) and myc4 (GK_491E10) were obtained from the ABRC or NASC, and identified by PCR with T-DNA specific and flanking primers (Supplementary Table 1 ). kix8-1 kix9-1 plants were obtained by crossing kix8 - 1 with kix9-1 plants and identified by PCR with primers of kix8-1F/1R and kix9-1F/1R (Supplementary Table 1 ). gif1 kix8-1 kix9-1 plants were obtained by crossing kix8-1 kix9-1 with gif1 plants and identified by PCR with primers of kix8-1F/1R, kix9-1F/1R and gif1-F/R (Supplementary Table 1 ). myc3 myc4 plants were obtained by crossing myc3 with myc4 plants and identified by PCR with primers of myc3-F/R and myc4F/R (Supplementary Table 1 ). gif1 myc3 myc4 plants were obtained by crossing myc3 myc4 with gif1 plants and identified by PCR with primers of myc3-F/R, myc4F/R and gif1-F/R (Supplementary Table 1 ). 35S : SAP plants were described before [23] . The ppd1 - 2 ppd2 - cr and ppd1 - cr ppd2 - 1 mutants were obtained by CRISPR-Cas9 mediated genome editing [27] . PPD2 - gRNA and PPD1 - gRNA was cloned into the pBluescript - AtU6 - SK vector, and then AtU6 - gRNA sequence was transferred to the pCAMBIA1300 - pYAO : Cas9 vector to generate pCAMBIA1300 - pYAO : Cas9 - AtU6 - gRNA constructs. The final constructs were transferred into ppd1 - 2 or ppd2 - 1 plants by agrobacterium tumefaciens-mediated transformation [50] . Transgenic plants were screened out with 30 μg ml −1 hygromycin. Genome-edited ppd1 - 2 ppd2 - cr and ppd1 - cr ppd2 - 1 mutants were identified by the sequencing of the PCR products with PPD1 and PPD2 specific primers (PPD1-CRIJD-F/R and PPD2-CRIJD-F/R) (Supplementary Fig. 1 , Supplementary Table 1 ). gif1 ppd1 - 2 ppd2 - cr plants were obtained by crossing ppd1 - 2 ppd2 - cr with gif1 plants. The gif1 and ppd1 - 2 mutations in gif1 ppd1 - 2 ppd2 - cr plants were identified by PCR with primers of gif1-F/R and ppd1-2F/R. The ppd2 - cr mutation in gif1 ppd1 - 2 ppd2 - cr plants were identified by the sequencing of the PCR products with PPD2 specific primers (PPD2-CRIJD-F/R) (Supplementary Table 1 ). The CDS of GIF1 was obtained from the total RNA of the Col-0 plants with FastQuant RT Super Mix kit (TIANGEN, KR108) and cloned into the Kpn I and Spe I sites of pMDC32 vector to generate pMDC32 - 35S : GIF1 constructs with EZfusion kit (Genera, GR6086). pMDC32 - 35S : GIF1 constructs were transferred into the Col-0 plants by agrobacterium tumefaciens-mediated transformation [50] . 35S : GIF1 transgenic plants were screened out with 30 μg ml −1 hygromycin. Seeds were sterilised with ethanol (75% v/v) for 3 min, bleach (10% v/v) for 15 min, and washed with sterilised water three times, and then plated to Murashige and Skoog (MS) medium. After storing in dark for 4 days at 4 °C, seeds were grown at 22 °C with 16 h light (28 W/6500 K)/8 h dark. Plant transformation and screen The transgenic plants were obtained by agrobacterium tumefaciens-mediated transformation [50] . Constructs were transferred into GV3101 agrobacterium cells. Agrobacterium cells were grown in LB medium containing 1% (m/v) Trypton, 0.5% (m/v) Yeast Extract, and 1% (m/v) NaCl (pH 7) at 28 °C overnight. Bacteria were pelleted and resuspended to 0.8 OD 600 concentration with the solution containing 0.22% (m/v) MS, 0.05% (v/v) Silwet L-77, 5% (m/v) sucrose, and 0.02% (m/v) MES (pH 5.7). Inflorescences of Col-0 plants were used for transformation. After transformation, plants were immediately covered with plastic bags and grew overnight before bags were removed. The transgenic plants were screened out with 30 μg ml −1 hygromycin. Morphological and cellular analysis Seeds were harvested from the third to seventh silique on the stem of plants. Cotyledons were harvested from the 8-day-old seedlings. Siliques were harvested at 14 DAF (days after flowering). Parameters of seeds, cotyledons, and siliques were measured by ImageJ software after photographing. For seed weight, 100 seeds were weighed at each experiment by Mettler Toledo XP6 (Mettler Toledo, Switzerland). As for seed integument observation, the stamens in the fourth flower on the stem of plants were removed before flowering. The plants were pollinated with their own pollens. The seeds were harvested at 0, 2, 4 and 6 DAP (days after pollination). Ovules from six siliques, which were from the fourth silique on the stem of six plants, were used for analysis. At least five representative ovules were analysed. Seeds from six siliques, which were from the fourth silique on the stem of six plants, were used for analysis. At least five representative seeds in a silique were used for analysis. Seeds were firstly cleared with FAA solution (90 mL 70% ethanol, 5 mL acetic acid, and 5 mL 37% formaldehyde), and then dealt with Hoyer’s solution (7.5 g gum arabic, 100 g chloral hydrate, 5 mL glycerol, 5 mL phenol, and 25 mL water) before used to observation under the differential interference contrast microscope (DIC, Leica DM2500). The integument cell number of seeds was counted in DIC. The integument length of seeds was matured by ImageJ. Subcellular localisation analysis The promotors of KIX8 (2,087 bp), KIX9 (1,714 bp), PPD1 (1,797 bp), PPD2 (2,153 bp), MYC3 (2,180 bp), MYC4 (2,132 bp), and GIF1 (2,337 bp) and their CDSs were cloned into the Asc I and Xba I sites of pMDC107 - GFP vector to generate KIX8pro : KIX8 - GFP , KIX9pro : KIX9 - GFP , PPD1pro : PPD1 - GFP, PPD2pro : PPD2 - GFP , MYC3pro : MYC3 - GFP , MYC4pro : MYC4 - GFP , and GIF1pro : GIF1 - GFP constructs with EZfusion kit (Genera, GR6086), respectively. The constructs of KIX8pro : KIX8 - GFP , KIX9pro : KIX9 - GFP , PPD1pro : PPD1 - GFP , PPD2pro : PPD2 - GFP , MYC3pro : MYC3 - GFP , MYC4pro : MYC4 - GFP , and GIF1pro : GIF1 - GFP were transferred into Col-0 plants by agrobacterium tumefaciens-mediated transformation. Transgenic plants were screened out with 30 μg ml −1 hygromycin. The GFP fluorescence in ovules and seeds was observed by the confocal microscopy (LSM710, Zeiss, Germany). Split luciferase complementation assays The CDSs of MYC2 , MYC3 and MYC4 were obtained from the total RNA of the Col-0 plants with FastQuant RT Super Mix kit (TIANGEN, KR108) and cloned into the Sal I site of pCAMBIA - split_nLUC vector with EZfusion kit (Genera, GR6086). The CDSs of KIX8 , KIX9 , PPD1 , and PPD2 were obtained from the total RNA of the Col-0 plants with FastQuant RT Super Mix kit (TIANGEN, KR108) and cloned into the Kpn I site of pCAMBIA - split_cLUC vector with EZfusion kit (Genera, GR6086). Split luciferase complementation assay was conducted as described previously [51] . Constructs were transferred into GV3101 agrobacterium cells. Agrobacterium cells were grown in LB medium containing 1% (m/v) Trypton, 0.5% (m/v) Yeast Extract, and 1% (m/v) NaCl (pH 7) at 28 °C to 0.8 OD 600 concentration. 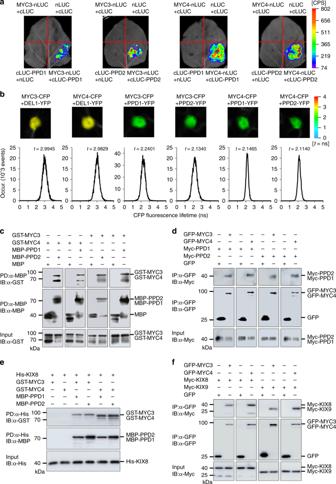Fig. 2: KIX8/9, PPD1/2, and MYC3/4 form a complex in Arabidopsis. aSplit luciferase complementation assays showing the interactions between PPD1/2 and MYC3/4. MYC3/4-nLUC and cLUC-PPD1/2 were coexpressed inN. benthamianaleaves. The luciferase activity was detected at 2 days later after infiltration.bThe FRET-FLIM assays showing that MYC3/4 interact with PPD1/2 inN. benthamianaleaves. CFP fluorescence lifetime was obtained at 2 days later after coinfiltrating with different combinations of35S:MYC3-CFP,35S:MYC4-CFP,35S:PPD1-YFP,35S:PPD2-YFP, and35S:DEL1-YFPconstructs.35S:DEL1-YFPwas used as a negative control.cPull-down analyses showing the interactions between PPD1/2 and MYC3/4 in vitro. GST-MYC3 and GST-MYC4 were incubated with MBP-PPD1, MBP-PPD2, and MBP, respectively. Proteins were pulled down by MBP-Trap-A agarose beads and detected by Western blot with anti-GST or anti-MBP antibody.dCo-immunoprecipitation analyses showing the interactions between PPD1/2 and MYC3/4 in Arabidopsis. Total protein extracts of35S:Myc-PPD1/2;35S:GFPand35S:Myc-PPD1/2;35S:GFP-MYC3/4plants were incubated with GFP-Trap agarose beads. Precipitates were detected by Western blot with anti-GFP or anti-Myc antibody.ePull-down analyses showing that PPD1/2 are required for the interactions between KIX8 and MYC3/4. His-KIX8 was incubated with GST-MYC3 or GST-MYC4 and MBP-PPD1 or MBP-PPD2. Proteins were pulled down by the Ni-NTA agarose beads and detected by Western blot with anti-GST, anti-MBP, or anti-His antibody.fCo-immunoprecipitation analyses showing that KIX8/9 and MYC3/4 are in a protein complex in Arabidopsis. Total protein extracts of35S:Myc-KIX8/9;35S:GFPand35S:Myc-KIX8/9;35S:GFP-MYC3/4plants were incubated with GFP-Trap agarose beads. Precipitates were detected by Western blot with anti-GFP or anti-Myc antibody. Bacteria were pelleted and resuspended to 0.5 OD 600 concentration with the solution containing 10 mM MES (pH 5.7), 10 mM MgCl 2 , and 150 mM Acetosyringone. The combinations of MYC2 - nLUC / cLUC - PPD1 / 2 , MYC2 - nLUC / cLUC - KIX8 / 9 , MYC3 - nLUC / cLUC - PPD1 / 2 , MYC3 - nLUC / cLUC - KIX8 / 9 , MYC4 - nLUC / cLUC - PPD1 / 2 , MYC4 - nLUC / cLUC - KIX8 / 9 , MYC2 / 3 / 4 - nLUC / cLUC , nLUC / cLUC - PPD1 / 2 and nLUC / cLUC - KIX8 / 9 were transferred into N. benthamiana leaves by agrobacterium tumefaciens-mediated transformation. The luciferase activity was detected 2 days later after infiltration. One millimolar luciferin (Sigma, 11626353001) was sprayed onto leaves, and the materials were kept in dark for 5 min. Images were obtained with CCD imaging apparatus (CHEMIPROHT 1300B/LND; Roper Scientific). FRET-FLIM analysis The CFP and YFP sequences were cloned into the Sac I site of pMDC32 vector to generate pMDC32 - CFP / YFP constructs with EZfusion kit (Genera, GR6086). The CDSs of MYC3 and MYC4 were obtained from the total RNA of the Col-0 plants with FastQuant RT Super Mix kit (TIANGEN, KR108) and cloned into the Sac I and Kpn I sites of pMDC32 - CFP construct to generate pMDC32 - MYC3 / MYC4 - CFP constructs with EZfusion kit (Genera, GR6086). The CDSs of PPD1 , PPD2 , and DEL1 were obtained from the total RNA of the Col-0 plants with FastQuant RT Super Mix kit (TIANGEN, KR108) and cloned into the Sac I and Kpn I sites of pMDC32 - YFP construct to generate pMDC32 - PPD1 / PPD2 / DEL1 - YFP constructs with EZfusion kit (Genera, GR6086). Constructs were transferred into GV3101 agrobacterium cells. Agrobacterium cells were grown in LB medium containing 1% (m/v) Trypton, 0.5% (m/v) Yeast Extract, and 1% (m/v) NaCl (pH 7) at 28 °C to 0.8 OD 600 concentration. Bacteria were pelleted and resuspended to 0.5 OD 600 concentration with the solution containing 10 mM MES (pH 5.7), 10 mM MgCl 2 , and 150 mM Acetosyringone. The different combinations of 35S : MYC3 - CFP , 35S : MYC4 - CFP , 35S : PPD1 - YFP , 35S : PPD2 - YFP and 35S : DEL1 - YFP constructs were coinfiltrated into N. benthamiana leaves by GV3101 agrobacterium cells. CFP fluorescence lifetime was obtained at 2 days later after coinfiltration by the confocal microscopy (LSM710, Zeiss, Germany) and TCSPC module and picosecond event timer (PicoQuant, Germany). Bimolecular fluorescence complementation assays The cYFP - MYC3 / 4 and nYFP - PPD1 / 2 constructs were generated by transferring the CDSs of MYC3 / 4 and PPD1 / 2 into the Xba I and SalI sites of pGWB414 - cYFP and pGWB414 - nYFP vectors with EZfusion kit (Genera, GR6086), respectively. Constructs were transferred into GV3101 agrobacterium cells. Agrobacterium cells were grown in LB medium containing 1% (m/v) Trypton, 0.5% (m/v) Yeast Extract, and 1% (m/v) NaCl (pH 7) at 28 °C to 0.8 OD 600 concentration. Bacteria were pelleted and resuspended to 0.5 OD 600 concentration with the solution containing 10 mM MES (pH 5.7), 10 mM MgCl 2 , and 150 mM Acetosyringone. The combinations of cYFP - MYC3 / nYFP - PPD1 / 2 , cYFP - MYC4 / nYFP - PPD1 / 2 , cYFP - MYC3 / 4 / nYFP , and cYFP / nYFP - PPD1 / 2 were coinfiltrated into N. benthamiana leaves by GV3101 agrobacterium cells. The YFP fluorescence was observed with the confocal microscope (LSM710, Zeiss, Germany) 2 days later after infiltration. 4′,6-diamidino-2-phenylindole (DAPI, Sigma, D9542) with 2 µg/ml was used to stain the nuclei. Pull-down assays The CDSs of MYC3 and MYC4 were obtained from the total RNA of the Col-0 plants with FastQuant RT Super Mix kit (TIANGEN, KR108) and cloned into the EcoR I site of pGEX4T1 - GST vector to generate GST - MYC3 / 4 constructs with EZfusion kit (Genera, GR6086). The CDSs of PPD1 and PPD2 were obtained from the total RNA of the Col-0 plants with FastQuant RT Super Mix kit (TIANGEN, KR108) and cloned into the BamH I site of pMALC2 - MBP vector to generate MBP - PPD1 / 2 constructs with EZfusion kit (Genera, GR6086). The CDSs of KIX8 and KIX9 were obtained from the total RNA of the Col-0 plants with FastQuant RT Super Mix kit (TIANGEN, KR108) and cloned into the Nco I site of pET24a - His vector to generate His - KIX8 / 9 constructs with EZfusion kit (Genera, GR6086). Pull-down assays were carried out as a previous study [52] . Constructs were transferred into E. coli BL21 (DE3) cells. All proteins were expressed in E. coli BL21 (DE3) with 0.5 mM Isopropyl β- d -1-thiogalactopyranoside (IPTG) at 28 °C for 4 h. BL21 (DE3) cells were pelleted and resuspended with the solution containing 50 mM HEPES (pH 7.5), 150 mM NaCl, 1 mM EGTA, 1% (v/v) Triton X-100, 10% (v/v) glycerol, and 1 mM PMSF. Proteins were obtained from bacteria after sonicating for 5 min (5 s on, 10 s stop) at 20 amplitude. The combinations of GST-MYC3/4, MBP-PPD1/2, and His-KIX8/9 proteins were incubated at 4 °C for 1 h and pulled down with anti-MBP agarose beads (NEB, E8037s) or Ni-NTA agarose beads (Invitrogen, R90115). Beads were washed 4 times with the solution containing 50 mM HEPES (pH 7.5), 150 mM NaCl, 1 mM EGTA, 0.5% (v/v) Triton X-100, 10% (v/v) glycerol, and 1 mM PMSF. Proteins were extracted with the solution containing 250 mM Tris-HCl (pH 6.8), 10% (w/v) SDS, 30% (v/v) glycerol, 5% (v/v) mercaptoethanol, 0.02% (m/v) bromophenol blue after boiling at 98 °C for 5 min. Proteins were detected by western blot with anti-GST (1:5000, Abmart, M20007), anti-His (1:2000, Abmart, M20001), or anti-MBP antibody (1:5000, Abmart, T40007). Co-immunoprecipitation The 35S : GFP - MYC2 / 3 / 4 constructs were generated by transferring the CDSs of MYC2 / 3 / 4 into the Asc I and Sal I sites of pMDC43 vector with EZfusion kit (Genera, GR6086). 35S : Myc - KIX8 / 9 and 35S : Myc - PPD1 / 2 constructs were generated by transferring the CDSs of KIX8 / 9 and PPD1 / 2 into the Kpn I site of pCambia1300 - 221 - Myc vector . 35S : GFP - MYC2 / 3 / 4 , 35S : Myc - KIX8 / 9 , and 35S : Myc - PPD1 / 2 transgenic Arabidopsis plants were obtained by agrobacterium tumefaciens-mediated transformation. 35S : Myc - PPD1 / 2 ; 35S : GFP - MYC2 / 3 / 4 , 35S : Myc - KIX8 / 9 ; 35S : GFP - MYC3 / 4 , 35S : Myc - PPD1 / 2 ; 35S : GFP , and 35S : Myc - KIX8 / 9 ; 35S : GFP plants were obtained by crossing 35S : Myc - PPD1 / 2 or 35S : Myc - KIX8 / 9 with 35S : GFP - MYC2 / 3 / 4 and 35S : GFP , respectively. The co-immunoprecipitation was conducted as described previously. Plants were ground with liquid nitrogen and proteins were dissolved with the buffer (50 mM Tris-HCl, 20% (v/v) glycerol, 150 mM NaCl, 2% (v/v) Triton X-100, 1 mM EDTA, 1× protease inhibitor cocktail, pH 7.5). The combinations of GFP, GFP-MYC2/3/4, Myc-KIX8/9, and Myc-PPD1/2 proteins were incubated at 4 °C for 1 h and pulled down with GFP-Trap agarose beads (Qualityard, QYA03914AAC). Beads were washed 4 times with the solution containing 50 mM Tris-HCl (pH 7.5), 20% (v/v) glycerol, 150 mM NaCl, 0.5% (v/v) Triton X-100, 1 mM EDTA, and 1× protease inhibitor cocktail. Proteins were extracted with the solution containing 250 mM Tris-HCl (pH 6.8), 10% (w/v) SDS, 30% (v/v) glycerol, 5% (v/v) mercaptoethanol, 0.02% (m/v) bromophenol blue after boiling at 98 °C for 5 min. 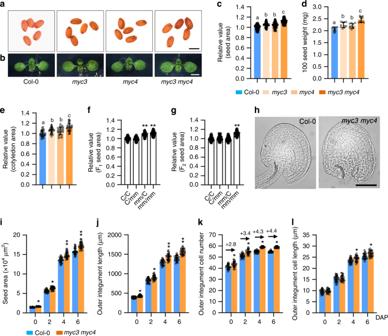Fig. 3:MYC3andMYC4act maternally to control seed development. a,bThe seeds (a) and 8-day-old seedlings (b) of Col-0,myc3,myc4, andmyc3 myc4.c–eThe relative seed area (c,n= 100), 100 seed weight (d,n= 10), and cotyledon area (e,n= 30) of Col-0,myc3,myc4andmyc3 myc4. Seeds from the third to seventh silique on the stem of six plants were used for analysis. Cotyledons from the 8-day-old seedlings were used for analysis.f,gThe relative area of F1seeds (f) and F2seeds (g) from the Col-0/Col-0 (C/C), Col-0/myc3 myc4(C/mm),myc3 myc4/Col-0 (mm/C), andmyc3 myc4/myc3 myc4(mm/mm) plants (n = 100).hOvules of Col-0 andmyc3 myc4plants at 0 DAP (days after pollination).i–lThe seed area (i), outer integument length (j), outer integument cell number (k), and outer integument cell length (l) of Col-0 andmyc3 myc4plants at 0, 2, 4, and 6 DAP (n = 33). Ovules and seeds from six siliques, which were from the fourth silique on the stem of six plants, were used for analysis. Scale bars, 0.5 mm (a), 0.2 cm (b), and 50 μm (h). Error bars represent ±SE. Different lowercase letters above the columns indicate the significant difference among different groups, one-way ANOVAP-values:P< 0.05. * indicates significant difference from the Col-0, one-way ANOVAP-values: *P< 0.05 and **P< 0.01. Proteins were detected by western blot with anti-Myc (1:5000, Abmart, M20002) or anti-GFP antibody (1:8000, Invitrogen, MA5-15256). qPCR and RNA-Seq analysis Total RNA was extracted according to the procedure of RNAprep pure kit (TIANGEN, DP439-H). The first cDNA was produced according to the procedure of FastQuant RT Super Mix kit (TIANGEN, KR108). qPCR was conducted with the SYBR Green І (ROCHE) by the realplex [2] (eppendorf). Data were normalised with ACTIN2 . For RNA-seq, the first pair of leaves from 9-day-old myc3 myc4 and ppd1 - 2 ppd2 - cr seedlings were harvested. The RNA extraction, sequencing, and analysis were conducted by Biomarker Technologies Corporation (China). Three biological replicates were performed for RNA-seq analyses. In brief, total RNA was extracted according to the procedure of RNeasy Plant Mini Kit (Qiagen). RNA-seq was performed with the Illumina HiSeq X platform (Illumina Inc., San Diego, CA) using 150-bp double-ended reads. The reads were aligned to the Arabidopsis reference genome (version TAIR10) using TopHat (version 2.0.12). P -values were adjusted using the Benjamini-Hochberg procedure. Differentially expressed genes were defined based on the P -values: P < 0.05. Dual-luciferase transient expression assay Dual-luciferase transient expression assays were carried out in the Arabidopsis protoplast. The CDSs of KIX8 , KXI9 , PPD1 , PPD2 , MYC3 , MYC4 , and TOPLESS were cloned into the Kpn I site of pCambia1300 - 221 - Myc vector to generate 35S : Myc - KIX8 , 35S : Myc - KIX9 , 35S : Myc - PPD1 , 35S : Myc - PPD2 , 35S : Myc - MYC3 , 35S : Myc - MYC4 , and 35S : Myc - TOPLESS constructs with EZfusion kit (Genera, GR6086). The 2337 bp sequence of GIF1 promoter was cloned into the Hind III site of pGreen II_0800 - LUC vector to generate the GIF1pro : LUC contruct with EZfusion kit (Genera, GR6086). Arabidopsis protoplast was isolated as described before. GIF1pro : LUC was cotransfected with different combinations of 35S : Myc - KIX8 , 35S : Myc - KIX9 , 35S : Myc - PPD1 , 35S : Myc - PPD2 , 35S : Myc - MYC3 , 35S : Myc - MYC4 , and 35S : Myc - TOPLESS into the Arabidopsis protoplast. Protoplasts were incubated at 23 °C for 36 h. LUC and REN luciferase activities were measured using the dual luciferase assay kit (Promega, E1500). The analysis was performed using the Luminoskan Ascent Microplate Luminometer (Thermo Fisher Scientific). Chromatin immunoprecipitation analysis In all, 1–4 DAF siliques of 35S : GFP , 35S : GFP - MYC3 ; myc3 , 35S : GFP - MYC4 ; myc4 , 35S : GFP - MYC3 ; myc3 ppd1 - 2 ppd2 - cr , 35S : GFP - MYC4 ; myc4 ppd1 - 2 ppd2 - cr , 35S : GFP - MYC3 ; myc3 kix8 - 1 kix9 - 1 , 35S : GFP - MYC4 ; myc4 kix8 - 1 kix9 - 1 , 35S : GFP - PPD1 ; ppd1 - 2 , 35S : GFP - PPD2 ; ppd2 - 1 , 35S : GFP - PPD1 ; ppd1 - 2 myc3 myc4 , 35S : GFP - PPD2 ; ppd2 - 1 myc3 myc4 , 35S : GFP - KIX8 ; kix8 - 1 , 35S : GFP - KIX9 ; kix9 - 1 , 35S : GFP - KIX8 ; kix8 - 1 myc3 myc4 and 35S : GFP - KIX9 ; kix9 - 1 myc3 myc4 were used for Chromatin extraction. The 35S : GFP - KIX8 ; kix8 - 1 , 35S : GFP - KIX9 ; kix9 - 1 , 35S : GFP - PPD1 ; ppd1 - 2 , 35S : GFP - PPD2 ; ppd2 - 1 , 35S : GFP - MYC3 ; myc3 and 35S : GFP - MYC4 ; myc4 plants with small seeds were used for the analysis (Supplementary Fig. 12 ). Chromatin immunoprecipitation analyses (ChIP-qPCR) were carried out as described before [53] . Siliques were cross-linked with the buffer (0.4 M sucrose, 15 mM PIPESl (pH 6.8), 1 mM EDTA, 1 mM PMSF, 1% (v/v) formaldehyde) and vacuumized for 15 min at room temperature. The cross-linking was stop by adding 2 M glycine to final concentration of 100 mM. Siliques were washed three times in sterile deionized water and ground to a fine powder with liquid nitrogen. Nuclei were isolation with the buffer (0.25 M sucrose, 15 mM PIPES (pH 6.8), 5 mM MgCl 2 , 60 mM KCl, 15 mM NaCl, 1 mM CaCl 2 , 1% (v/v) Triton X-100, 2.5% (v/v) Ficoll 400, 3.12 µL/mL mercaptoethanol, 1× protease inhibitor coctail). Chromatins were extracted with cold nuclei lysis buffer containing 50 mM Tris-HCl (pH 8), 10 mM EDTA, 1% (m/v) SDS after centrifugation at 4 °C × 3000 g for 20 min, and sonicated five times for 10 s at power 6. Chromatins were incubated with ChIP anti-GFP antibody (1:100, Invitrogen, MA5-15256) at 4 °C overnight. 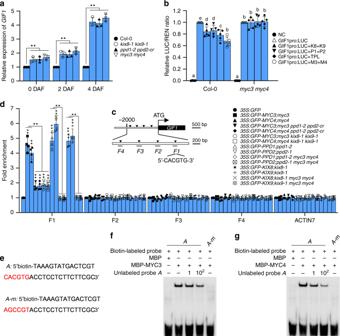Fig. 4: The KIX-PPD-MYC complex associates with the promoter ofGIF1and represses its expression. aThe relative expression levels ofGIF1in the 0, 2 and 4 DAF (days after flowering) siliques of Col-0,kix8-1 kix9-1,ppd1-2 ppd2-crandmyc3 myc4were detected by qPCR (n= 3). Data was normalised withACTIN2.bThe LUC activity ofGIF1pro:LUCfrom the transient expression analysis in the Col-0 andmyc3 myc4protoplast (n= 5).GIF1pro:LUCwas cotransfected with different combinations of35S:Myc-KIX8(K8),35S:Myc-KIX9(K9),35S:Myc-PPD1(P1),35S:Myc-PPD2(P2),35S:Myc-MYC3(M3),35S:Myc-MYC4(M4), and35S:Myc-TPL(TPL) into the Col-0 andmyc3 myc4protoplast. The LUC and REN luciferase activities ofGIF1pro:LUCwere measured 40 h later after transfection. NC (pGreen II_0800-LUC) was used as a negative control.cThe schematic diagram ofGIF1promoter containing a typical G-box (5′-CACGTG-3′) sequence inF1fragment.F1-F4represent DNA fragments used for ChIP-qPCR analysis.dChIP-qPCR assays showing that KIX8/9 and PPD1/2 associate with the promoter ofGIF1by MYC3/4 in Arabidopsis (n= 4). Chromatin from 1 to 4 DAF siliques of35S:GFP,35S:GFP-MYC3;myc3,35S:GFP-MYC4;myc4,35S:GFP-MYC3;myc3ppd1-2 ppd2-cr,35S:GFP-MYC4;myc4 ppd1-2 ppd2-cr,35S:GFP-MYC3;myc3 kix8-1kix9-1,35S:GFP-MYC4;myc4 kix8-1kix9-1,35S:GFP-PPD1;ppd1-2,35S:GFP-PPD2;ppd2-1,35S:GFP-PPD1;ppd1-2 myc3 myc4,35S:GFP-PPD2;ppd2-1 myc3 myc4,35S:GFP-KIX8;kix8-1,35S:GFP-KIX9;kix9-1,35S:GFP-KIX8;kix8-1 myc3 myc4and35S:GFP-KIX9;kix9-1 myc3 myc4were incubated with ChIP anti-GFP antibody and precipitated by ChIP protein A + G magnetic beads. The enrichment of fragments was determined by qPCR. The35S:GFPplants acted as a control. TheACTIN7promoter was used as a negative control.eThe sequence ofAandA-mprobes for EMSA analysis.f,gThe associations of MBP-MYC3 (g) and MBP-MYC4 (i) with the promoter ofGIF1were detected by EMSA. 5′-biotin-A/A-mprobes were incubated with MBP or MBP-MYC3/4 and detected by ChIP western blot with the anti-biotin antibody. Error bars represent ±SE. Asterisk indicates significant difference, one-way ANOVAP-values: **P< 0.01. Different lowercase letters above the columns indicate the significant difference among different groups, one-way ANOVAP-values:P< 0.05. 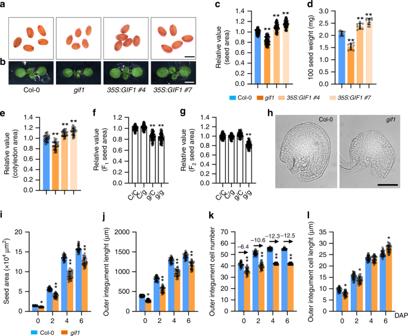Fig. 5:GIF1acts maternally to control seed development. a,bThe seeds (a) and 8-day-old seedlings (b) of Col-0,gif1,35S:GIF1 #4, and35S:GIF1 #7.c–eThe relative seed area (c,n= 100), 100 seed weight (d,n= 10), and cotyledon area (e,n= 30) of Col-0,gif1,35S:GIF1 #4, and35S:GIF1 #7. Seeds from the third to seventh silique on the stem of six plants were used for analysis. Cotyledons from the 8-day-old seedlings were used for analysis.f,gThe relative area of F1seeds (f) and F2seeds (g) from Col-0/Col-0 (C/C), Col-0/gif1(C/g),gif1/Col-0 (g/C), andgif1/gif1(g/g) plants (n= 100).hThe Mature ovule of Col-0 andgif1plants at 0 DAP (days after pollination).i–lThe seed area (i), outer integument length (j), outer integument cell number (k), and outer integument cell length (l) of Col-0 andgif1plants at 0, 2, 4, and 6 DAP (n = 33). Ovules and seeds from six siliques, which were from the fourth silique on the stem of six plants, were used for analysis. Scale bars, 0.5 mm (a), 0.2 cm (b), and 50 μm (h). Error bars represent ±SE. Different lowercase letters above the columns indicate the significant difference among different groups, one-way ANOVAP-values:P< 0.05. Asterisk indicates significant difference from the Col-0, one-way ANOVAP-values: *P< 0.05 and **P< 0.01. The coupled-chromatin fragments were pulled down by ChIP protein A + G magnetic beads (1:50, Magna, 16-663) at 4 °C for 4 h. The beads were washed for 5 min each time at 4 °C with 1 ml of each of the following buffers: 2 times with low salt wash buffer (150 mM NaCl, 20 mM Tris–HCl (pH 8), 0.2% (m/v) SDS, 0.5% (v/v) Triton X-100, and 2 mM EDTA), two times with high salt wash buffer (500 mM NaCl, 20 mM Tris–HCl (pH 8), 0.2% (m/v) SDS, 0.5% (v/v) Triton X-100, and 2 mM EDTA), two times with LiCl wash buffer (0.25 M LiCl, 1% (m/v) sodium deoxycholate, 10 mM Tris–HCl (pH 8), 1% (v/v) NP-40, and 1 mM EDTA), and two times with TE buffer (1 mM EDTA and 10 mM Tris–HCl pH 8). DNA was extracted from the beads with elution buffer containing 0.5% (m/v) SDS and 0.1 M NaHCO 3 at 65 °C for 15 min and reversely cross-linked with 192 mM NaCl at 65 °C for overnight. 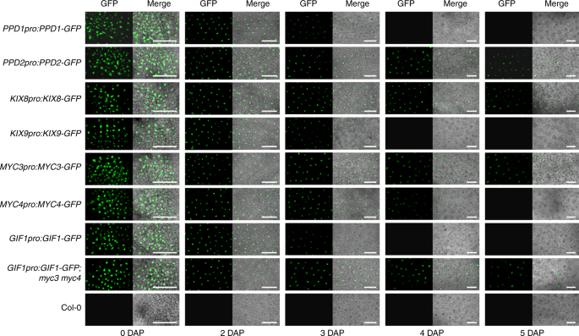Fig. 6: Expression patterns ofKIX8,KIX9,PPD1,PPD2,MYC3,MYC4, andGIF1in epidermal cells of the outer integuments during seed development. The promotors ofKIX8(2,087 bp),KIX9(1,714 bp),PPD1(1,797 bp),PPD2(2,153 bp),MYC3(2,180 bp),MYC4(2,132 bp), andGIF1(2,337 bp) and their CDSs were cloned into thepMDC107-GFPvector to generateKIX8pro:KIX8-GFP,KIX9pro:KIX9-GFP,PPD1pro:PPD1-GFP, PPD2pro:PPD2-GFP,MYC3pro:MYC3-GFP,MYC4pro:MYC4-GFP, andGIF1pro:GIF1-GFPconstructs, respectively. GFP fluorescence from the outer integuments of seeds was observed during seed development. DAP days after pollination. Scale bars = 25 μm. 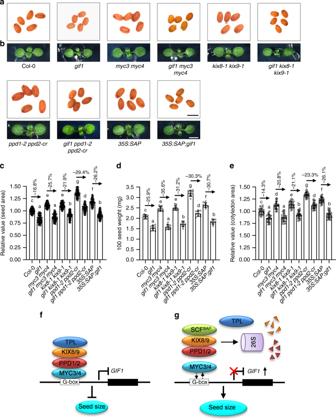Fig. 7: GIF1 acts genetically with the KIX-PPD-MYC complex to control seed size. a,bThe seeds (a) and 8-day-old seedlings (b) of Col-0,gif1,myc3 myc4,gif1 myc3 myc4,kix8-1 kix9-1,gif1 kix8-1 kix9-1,ppd1-2 ppd2-cr,gif1 ppd1-2 ppd2-cr,35S:SAP, and35S:SAP;gif1plants.c–eThe relative seed area (c,n= 100), 100 seed weight (d,n= 10), and cotyledon area (e,n= 30) of Col-0,gif1,myc3 myc4,gif1 myc3 myc4,kix8-1 kix9-1,gif1 kix8-1 kix9-1,ppd1-2 ppd2-cr,gif1 ppd1-2 ppd2-cr,35S:SAP, and35S:SAP;gif1plants.fThe TPL-KIX-PPD-MYC complex associates with the G-box sequence ofGIF1promoter and represses its expression.gThe transcriptional repression ofGIF1is relieved by SAP modulating the KIX-PPD module for 26S proteasome degradation. Without the KIX-PPD complex, the binding ability of MYC3/4 with the promoter ofGIF1is decreased and theGIF1expression is increased. Seeds from the third to seventh silique on the stem of six plants were used for analysis. Cotyledons from the 8-day-old seedlings were used for analysis. Scale bars, 0.5 mm (a) and 0.2 cm (b). Error bars represent ±SE. Different lowercase letters above the columns indicate the significant difference among different groups, one-way ANOVAP-values:P< 0.05. Proteins were removed with equal volume of phenol/chloroform/isoamyl alcohol (25:24:1). DNA was precipitated with 2.5 volume of 100% ethanol, 1/10 volume of 3 M sodium acetate (pH 5.2), and dissolved to TE buffer containing 1 mM EDTA and 10 mM Tris–HCl (pH 8). qPCR analysis was used to detected the enrichment of the chromatin fragments. 35S : GFP plants were used as the control. The promoter of ACTIN7 was used as a negative control. Electrophoretic mobility shift assay Electrophoretic mobility shift assay (EMSA) was performed according to the procedure of EMSA kit (Thermo). The CDSs of MYC3 and MYC4 were cloned into the pMALC2 - MBP vector to generate MBP - MYC3 and MBP - MYC4 constructs, respectively. Proteins were expressed in E. coli BL21 (DE3) with 0.5 mM Isopropyl β-D-1-thiogalactopyranoside (IPTG) at 28 °C for 4 h. BL21 (DE3) cells were pelleted at 4 °C × 5000 g for 15 min and resuspended with the solution containing 50 mM HEPES (pH 7.5), 150 mM NaCl, 1 mM EGTA, 1% (v/v) Triton X-100, 10% (v/v) glycerol, and 1 mM PMSF. Proteins were obtained from bacteria after sonicating for 5 min (5 s on, 10 s stop) at 20 amplitude. The biotin-labelled and unlabelled probes were synthesised and incubated with MBP, MBP-MYC3, or MBP-MYC4 at room temperature for 20 min. Proteins were purified with anti-MBP agarose beads (NEB, E8037s). The interactions were detected with an anti-biotin antibody (1:3000, Invitrogen, 03-3720). Reporting summary Further information on research design is available in the Nature Research Reporting Summary linked to this article.